The antimicrobial peptide LL37 is a T-cell autoantigen in psoriasis Psoriasis is a common T-cell-mediated skin disease with 2–3% prevalence worldwide. Psoriasis is considered to be an autoimmune disease, but the precise nature of the autoantigens triggering T-cell activation remains poorly understood. Here we find that two-thirds of patients with moderate-to-severe plaque psoriasis harbour CD4 + and/or CD8 + T cells specific for LL37, an antimicrobial peptide (AMP) overexpressed in psoriatic skin and reported to trigger activation of innate immune cells. LL37-specific T cells produce IFN-γ, and CD4 + T cells also produce Th17 cytokines. LL37-specific T cells can infiltrate lesional skin and may be tracked in patients blood by tetramers staining. Presence of circulating LL37-specific T cells correlates significantly with disease activity, suggesting a contribution to disease pathogenesis. Thus, we uncover a role of LL37 as a T-cell autoantigen in psoriasis and provide evidence for a role of AMPs in both innate and adaptive immune cell activation. Psoriasis is a very common inflammatory skin disease characterized by scaly erythematous plaques that may cover large body areas [1] , [2] . T cells infiltrate the skin and secrete IFN-γ and Th17 cytokines [3] , [4] , [5] , [6] that initiate the typical abnormal keratinocyte proliferation [6] , [7] , [8] , [9] . Despite the undisputable evidence of the role of T cells [8] and their secreted products [4] , [5] , [6] , [7] in psoriasis pathogenesis, the nature of the autoantigens that trigger T-cell activation still remains unclear. Psoriasis is characterized by an aberrant activation/maturation of dendritic cells (DCs) that stimulate autoimmune T cells in lesional skin and lymphoid organs [10] , [11] . An antimicrobial peptide (AMP) overexpressed in psoriatic skin has been suggested to play a role in this process [12] , [13] , [14] , [15] . This peptide, called LL37, is a cationic peptide that provides an important antimicrobial defense mechanism of damaged skin [12] . LL37 forms complexes with extracellular self-nucleic acids (present in lesional skin as the result of inflammatory process and associated cell damage) and allow entry of these nucleic acids into intracellular compartments containing TLR7/8/9 or cytosolic DNA sensors [13] , [14] , [15] . The chronic overexpression of LL37 induces sustained nucleic acid-mediated activation of these receptors, leading to maturation of DCs. However, whether LL37 also directly stimulate T cells serving as an autoantigen presented by maturing DCs to T cells is currently unknown. Our results show that LL37 is indeed recognized as an autoantigen by circulating T cells of 46% of psoriasis patients and more frequently in moderate-to-severe psoriasis (in up to 75% of patients with Psoriasis Activity Severity Index (PASI)>10). LL37-specific T cells produce pathogenic cytokines, including IL-17, and can be tracked in patient blood by tetramer staining. Thus we present here evidence that LL37 can act as an autoantigen for T cells and represents the first example of an AMP stimulating both innate [13] , [14] , [15] and adaptive immune cells in autoimmune settings. LL37 frequently induces proliferation of psoriatic T cells LL37 is strongly expressed in both dermis and epidermis of psoriatic skin lesions, mainly released by infiltrating neutrophils and expressed by keratinocytes, respectively [12] , [13] , [14] , [15] ( Supplementary Fig. 1 ). As psoriatic T cells can be stimulated by LL37-activated DCs and migrate into the epidermis to recognize an autoantigen expressed by keratinocytes, we asked whether LL37 would also serve as an autoantigen broadly expressed in psoriatic skin. To address this question we first investigated whether circulating psoriatic T cells would respond to LL37 by stimulating peripheral blood mononuclear cells (PBMCs) with 10 μg ml −1 of LL37 or scrambled LL37 (GL37) and measuring T-cell proliferation by BrdU-incorporation in CD3 + cells. The following control donors were tested in the same way: healthy donors, patients with scleroderma, reported to express elevated LL37 levels in their skin [16] , atopic dermatitis, as irrelevant inflammatory skin disease and erysipelas, as infectious skin disease ( Fig. 1a ). Total CD3 + cells from 24 out of 52 psoriasis patients (46%) proliferated to LL37 ( Fig. 1b and Supplementary Fig. 2a ) and produced IFN-γ ( Fig. 1c ), but none of the control individuals did. 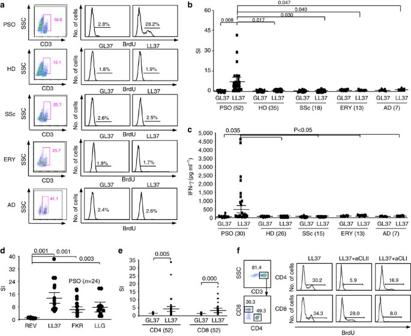Figure 1: Circulating T cells of psoriasis patients proliferate and produce IFN-γ in response to LL37 in a HLA-dependent manner. (a,b) BrdU incorporation by CD3+cells of psoriasis patients (PSO), healthy donors (HD), scleroderma (SSc), erysipela (ERY) and atopic dermatitis (AD) patients, stimulated for 6 days with LL37 or GL37. Percentage of BrdU+CD3+T cells was evaluated by flow cytometry and is given in the representative plots (a). Cumulative data are reported in (b) as stimulation indexes (SI) defined as BrdU incorporation of peptide-stimulated cells over untreated cells. Number of individuals tested are indicated in brackets. Values of SI>3 were considered positive. (c) IFN-γ released measured by ELISA by PBMCs stimulated as in (a) for 3 days. Number of patients and controls tested are reported in brackets. (d) BrdU incorporation by CD3+cells of PSO patients (n=24) on a 6-day stimulation of PBMCs with LL37 and control peptides. (e) BrdU incorporation by CD3+CD4+(CD4) or CD3+CD8+(CD8) cells on a 6-day stimulation of PBMCs of PSO patients (n=52) with LL37 or GL37. For all data inb–ehorizontal bars represent the mean, vertical bars s.e.m.,Pvalues by Student’st-test for paired samples (to compare response to LL37 or LL37 peptides FKR or LLG in psoriasis patients to control peptide GL37 in the same patient) or ANOVA for unpaired samples (to compare response to LL37 among each group of individuals tested). (f) PBMCs of PSO patients were stimulated with LL37 in the presence/absence of blocking antibodies against either HLA ClassI (aCLI) or HLA ClassII (aCLII). BrdU incorporation was used to assess proliferation of gated CD3+CD4+(CD4) or CD3+CD8+(CD8) cells. Representative flow cytometry plots and histograms are shown. Percent of positivity for BrdU is indicated. Figure 1: Circulating T cells of psoriasis patients proliferate and produce IFN-γ in response to LL37 in a HLA-dependent manner. ( a , b ) BrdU incorporation by CD3 + cells of psoriasis patients (PSO), healthy donors (HD), scleroderma (SSc), erysipela (ERY) and atopic dermatitis (AD) patients, stimulated for 6 days with LL37 or GL37. Percentage of BrdU + CD3 + T cells was evaluated by flow cytometry and is given in the representative plots ( a ). Cumulative data are reported in ( b ) as stimulation indexes (SI) defined as BrdU incorporation of peptide-stimulated cells over untreated cells. Number of individuals tested are indicated in brackets. Values of SI>3 were considered positive. ( c ) IFN-γ released measured by ELISA by PBMCs stimulated as in ( a ) for 3 days. Number of patients and controls tested are reported in brackets. ( d ) BrdU incorporation by CD3 + cells of PSO patients ( n =24) on a 6-day stimulation of PBMCs with LL37 and control peptides. ( e ) BrdU incorporation by CD3 + CD4 + (CD4) or CD3 + CD8 + (CD8) cells on a 6-day stimulation of PBMCs of PSO patients ( n =52) with LL37 or GL37. For all data in b – e horizontal bars represent the mean, vertical bars s.e.m., P values by Student’s t -test for paired samples (to compare response to LL37 or LL37 peptides FKR or LLG in psoriasis patients to control peptide GL37 in the same patient) or ANOVA for unpaired samples (to compare response to LL37 among each group of individuals tested). ( f ) PBMCs of PSO patients were stimulated with LL37 in the presence/absence of blocking antibodies against either HLA ClassI (aCLI) or HLA ClassII (aCLII). BrdU incorporation was used to assess proliferation of gated CD3 + CD4 + (CD4) or CD3 + CD8 + (CD8) cells. Representative flow cytometry plots and histograms are shown. Percent of positivity for BrdU is indicated. Full size image To ensure that T-cell activation by LL37 was sequence dependent and independent of its adjuvant activity, we next used either the inverse LL37 sequence (REV), which retains adjuvant activity but lacks correct LL37 sequence, or two LL37 fragments, FKR (C-term) and LLG (N-term), which do not retain adjuvant activity but have a correct sequence ( Supplementary Fig. 2b ). T cells proliferated to FKR and/or LLG ( Fig. 1d ), but not to REV, confirming sequence specificity of LL37-directed T-cell responses. We detected LL37-specific T cells of both CD4 + and CD8 + phenotype ( Fig. 1e,f ). In 13 out 24 LL37-reponder patients (54%) exclusively CD4 + T cells proliferated; both CD4 + and CD8 + T cells proliferated in 7 (29.1%) and exclusively CD8 + T cells responded in 4 patients (17.7%). Blocking HLA-ClassII and/or -ClassI significantly reduced proliferation of CD4 + and CD8 + T cells, respectively ( Fig. 1e,f ; Supplementary Fig. 2c ). HLA blocking also reduced IFN-γ production ( Supplementary Fig. 2d ). In patients with both CD4 + and CD8 + T-cell responses inhibition of the CD4 + or CD8 + subset activation significantly affected activation of the complementary subset ( Supplementary Fig. 1c , lower panels), which suggests an intimate cooperation of CD4 + and CD8 + T cells during LL37-mediated activation in vivo . To investigate whether psoriatic T cells were exclusively responding to LL37, we stimulated PBMCs with the keratinocyte-derived human-β-defensin2 (HBD2), or the neutrophil-derived α-defensins (HNP 1-3 ), also overexpressed in psoriasis [17] . We detected no significant responses, suggesting T-cell activation is not a broad feature of AMPs ( Supplementary Fig. 3 ). We also tested reactivity to keratins, as these proteins were identified as autoantigens in a subset of psoriasis patients [18] , [19] , [20] , [21] , [22] . In keeping with the literature [18] , [19] , [20] , [21] , [22] , we detected reactivity to Keratins that was statistically significant for Keratin17 ( Supplementary Fig. 3 , lefts panels). Six out of 23 patients tested responded to Keratin17 (26%) and two to Keratin6 (8.7%), respectively. Keratin-specific reactivity was only observed in patients who responded to LL37 with CD4 + T cells (6 out of 15 LL37-reponders, 40%, Supplementary Fig. 3a , left panel). To map LL37-T-cell-epitopes we used overlapping LL37 peptides of 13–15 amino acids (aa) or 9–10 aa to depict CD4 + or CD8 + T-cell responses, respectively ( Supplementary Fig. 4 ). A variety of LL37 epitopes stimulated proliferation, with peptides P1, P4, P6 and P7 being most frequently, but not exclusively immunogenic. In patients responding with CD8 + T cells, LL37 peptides of 9–10 aa elicited proliferation, suggesting that activation of CD8 + T cells by LL37 is not the result of bystander activation of CD4 + T cells ( Supplementary Fig. 4b ). To explain the high frequency of LL37-induced proliferation of psoriatic T cells we utilized available algorithms (see Methods) to search for ‘HLA-binding motifs’ [23] within LL37 sequence. These predictions revealed that LL37 harbours multiple ‘binding motifs’ for HLA-DR and ClassI-alleles, consistent with the observed broad LL37-peptide-specificity of psoriatic T cells. In particular, HLA-DR binding prediction showed that LL37 epitopes might bind frequently expressed HLA-DR alleles ( Supplementary Fig. 5 ). Of note, number of suitable binding motifs for HLA-DR alleles in the HBD2 and HNP1-3 sequences was lower than that predicted for LL37 sequence [24] . Therefore, we selected the three most frequently expressed HLA-DR molecules in Caucasians [25] , such as DR1, DR4 and DR11, and performed HLA-binding assays ( Supplementary Fig. 6a ). Some LL37 peptides were indeed good binder for these HLA alleles. As the frequency of HLA-ClassI allele Cw6*02 is higher in psoriasis as compared with unaffected individuals [26] , [27] , [28] , we assessed binding of LL37 peptides to Cw6*02 by MHC-refolding assays. Five LL37 sequences efficiently stabilized soluble Cw6*02-molecules, revealing consistent binding capacity ( Supplementary Fig. 6b ). LL37-reactive T cells correlate with severe disease As shown above, IFN-γ was detected in primary cultures from all patients proliferating to LL37. Next, we checked whether LL37-specific T cells also produced other cytokines. By using ELISA assays, IL-22 was detected in 45% of LL37-responders, IL-21 in 21% and IL-17 in 13% ( Fig. 2a ; Supplementary Fig. 7a ). Only one patient (5%) produced IL-10; IL-4 was undetectable. Detection by ELISA could, however, underestimate cytokine production, as only a small fraction of T cells proliferated to LL37 in primary culture conditions. Therefore, we analysed cytokines by intracellular staining in the T cells incorporating BrdU as the result of LL37 stimulation. BrdU + CD3 + cells contained mainly IFN-γ + T cells, that may coproduce IL-22, IL-21 and IL-17. We also observed small populations of IFN-γ − cells producing exclusively IL-22, IL-21 and IL-17 ( Supplementary Fig. 7b ). Also, using intracellular cytokine detection, we found higher percentages of LL37-responder T cells producing IL-17 as compared with ELISA tests (75%) ( Supplementary Fig. 7b–d ). When using PBMCs of healthy donors we did not detect any significant upregulation of IL-17 in response to LL37 ( Supplementary Fig. 7c,d ). A higher percentage of expression by LL37-proliferating T cells was also appreciated for IL-21 (71%) compared with ELISA detection, whereas we confirmed data on IL-22 (45%) and IFN-γ (100%) production. 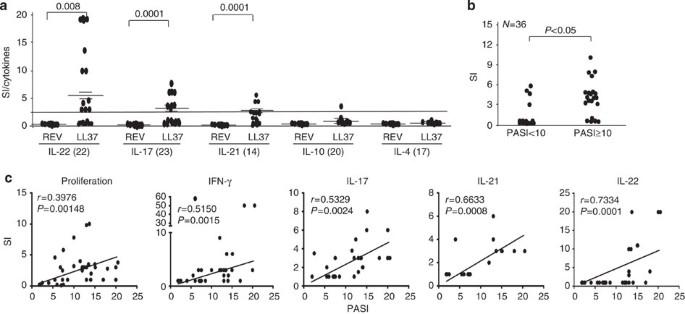Figure 2: LL37-reactive T cells produce Th17 cytokines and their detection correlates with disease severity. (a) Peripheral T cells of psoriatic patients were stimulated with either LL37 or REV peptide. IL-22 was measured after 3 days in culture supernatants by ELISA, other cytokines were measured by intracellular staining after 6-day culture with LL37 or REV peptide on gated BrdU+T cells. For all cytokines results are given as stimulation indexes (SI/cytokines, see Methods). Horizontal bars represent the mean, vertical bars are the s.e.m.Pvalues by Student’st-test for paired sample. (b) LL37-induced T-cell proliferation in psoriasis patients with mild disease (PASI score <10,n=16) and patients with moderate-to-severe disease (PASI score >10,n=20). Proliferation is indicated as SI. Values ≥3 were considered positive. Total number of patients is indicated.Pvalue by Student’st-test for unpaired samples. (c) Levels of LL37-specific T-cell proliferation and cytokine production plotted against psoriatic disease activity score (PASI). Statistical correlation was determined using two-tailed Spearman’s rank correlation test. The correlation coefficient (r) and significance (P) are indicated in each panel. Figure 2: LL37-reactive T cells produce Th17 cytokines and their detection correlates with disease severity. ( a ) Peripheral T cells of psoriatic patients were stimulated with either LL37 or REV peptide. IL-22 was measured after 3 days in culture supernatants by ELISA, other cytokines were measured by intracellular staining after 6-day culture with LL37 or REV peptide on gated BrdU + T cells. For all cytokines results are given as stimulation indexes (SI/cytokines, see Methods). Horizontal bars represent the mean, vertical bars are the s.e.m. P values by Student’s t -test for paired sample. ( b ) LL37-induced T-cell proliferation in psoriasis patients with mild disease (PASI score <10, n =16) and patients with moderate-to-severe disease (PASI score >10, n =20). Proliferation is indicated as SI. Values ≥3 were considered positive. Total number of patients is indicated. P value by Student’s t -test for unpaired samples. ( c ) Levels of LL37-specific T-cell proliferation and cytokine production plotted against psoriatic disease activity score (PASI). Statistical correlation was determined using two-tailed Spearman’s rank correlation test. The correlation coefficient (r) and significance ( P ) are indicated in each panel. Full size image Next we correlated responses to LL37 with disease status, measured by the PASI (see Methods). Fifteen out of 20 patients (75%) with PASI>10 responded to LL37, whereas positive responses were present in 4 out of 16 patients with PASI<10 (25%) ( Fig. 2b ). Proliferation and IFN-γ, IL-17, IL-22 and IL-21, but not IL-10 levels, significantly correlated with PASI, according to Pearson’s analysis ( Fig. 2c ). Interestingly, K statistics [29] revealed that association between presence of pathogenic cytokines and moderate-to-severe disease (PASI>10) was the strongest for IL-17, key pathogenic cytokine in psoriasis [5] , [6] , [7] , [30] ( Supplementary Table 1 ). Thus, LL37-specific T cells produced Th1 cytokines and a small minority also produced Th17 cytokines and their presence was associated with moderate-to-severe disease, suggesting a contribution to pathogenic events of LL37-specific T-cell responses. LL37-specific T cells are restricted by various HLA alleles To assess HLA restriction of LL37-specific T cells, we isolated T-cell lines from psoriasis patients. Two CD4 + T-cell lines (PSO4-1 and PSO4-2) derived from a HLA-DR11 + /DR4 + patient with PASI=18 recognized LL37 in the context of DR11 and DR4 (PSO4-1) or DR11 only (PSO4-2). CD4 + T-cell lines (PSO17-1 and PSO17-2) derived from a HLA-DR11 + /DR16 + patient with PASI=5 were also DR11-restricted. One CD4 + T-cell line (PSO8-1) derived from a HLA-DR7 + /DR16 + patient with PASI=20 was restricted by both HLA-DR7 and DR16 ( Fig. 3a ). All CD4 + T-cell lines produced IFN-γ, IL-17, IL-22 and/or IL-21. Surprisingly, PSO17-2 line also produced IL-4, IL-5 and IL-13 ( Fig. 3b ). 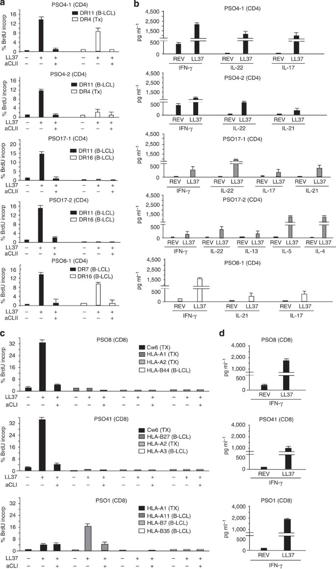Figure 3: Characterization and HLA restriction of LL37-specific T-cell lines of psoriasis patients. (a,c) Psoriatic CD4+T-cell lines PSO4-1, PSO4-2, PSO17-1, PSO7-2 and PSO8-1 (a), and CD8+T-cell lines PSO8, PSO41 and PSO1 (c) were cultured for three days with either unpulsed or LL37-loaded irradiated HLA-matched B-LCLs or transfectants (TX) in the presence/absence of (a) anti-HLA ClassII (aCLII) (for CD4+T-cell lines) or (c) anti-HLA ClassI (aCLI) (for CD8+T-cell lines) antibodies. Cytokine secretion was analysed in the culture supernatants by ELISA at day2 (b,d). In all panels the three experiments mean±s.e.m. are reported. Figure 3: Characterization and HLA restriction of LL37-specific T-cell lines of psoriasis patients. ( a , c ) Psoriatic CD4 + T-cell lines PSO4-1, PSO4-2, PSO17-1, PSO7-2 and PSO8-1 ( a ), and CD8 + T-cell lines PSO8, PSO41 and PSO1 ( c ) were cultured for three days with either unpulsed or LL37-loaded irradiated HLA-matched B-LCLs or transfectants (TX) in the presence/absence of ( a ) anti-HLA ClassII (aCLII) (for CD4 + T-cell lines) or ( c ) anti-HLA ClassI (aCLI) (for CD8 + T-cell lines) antibodies. Cytokine secretion was analysed in the culture supernatants by ELISA at day2 ( b , d ). In all panels the three experiments mean±s.e.m. are reported. Full size image We also obtained CD8 + T-cell lines from three patients with severe psoriasis (PASI>10). As HLA-Cw6*02 is strongly associated with psoriasis, and in particular with Type I psoriasis [26] , [27] , [28] , and LL37 peptides were identified as Cw6*02 binders, we tested Cw6*02 restriction. Two out of two CD8 + T-cell lines from Cw6*02 + patients exhibited consistent proliferative response to LL37-pulsed Cw6*02-expressing transfectants. No restriction to other ClassI alleles expressed by the patients was detectable ( Fig. 3c ). The restriction element of a third line (PSO1, from a Cw6*02 − patient) was HLA-A11. Thus, Cw6*02 could perform LL37 presentation to CD8 + T cells, but other alleles might have similar ability. All CD8 + T cells produced significant amounts of IFN-γ ( Fig. 3d ) and negligible Th17/Th2 cytokines. Epitope mapping of LL37-specific T cells showed that CD4 + T-cell lines, PSO4-1 (and PSO4-2, not shown) recognized peptide P4 presented by DR11 ( Fig. 4a,b ); PSO17-1 (and PSO17-2, not shown) recognized peptide P6 presented by DR11 ( Fig. 4c,d left panels); PSO8-1 recognized P4 presented by both DR7 and DR16 and, at low avidity, P6 in association with DR7 ( Fig. 4e,f left panels). Among CD8 + T-cell lines, PSO8 recognized peptides P7 and P6 ( Fig. 4g ) and, more precisely, the short LL37-peptide P7s (and to a lower extend the overlapping P6s) ( Fig. 4h , left panels). The second Cw6*02-restricted line PSO41 recognized P5s. Similar data were obtained by using CD4 + and CD8 + T-cell clones generated from PSO17, PSO8-1 and PSO8 lines ( Fig. 4c–h , right panels), although the CD4 + T-cell clone derived from PSO8-1 (PSO8-1 clone4) recognized only the LL37 C-term part (P6/P7) ( Fig. 4f , right panels). Thus, the fine characterization of LL37-directed T-cell responses indicates that multiple epitopes of LL37 sequence are immunogenic and that these epitopes can be presented by several HLA alleles. This is in accordance with HLA ‘binding motif’ predictions. 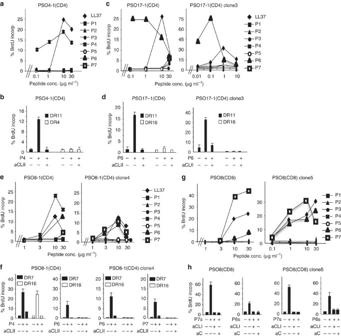Figure 4: Epitope mapping of LL37-specific T-cell lines and clones of psoriasis patients. (a,c,e,g) Percentage of BrdU incorporation in psoriatic CD4+T-cell lines PSO4-1 (a), PSO17-1 line, PSO17-1 clone3 (c), PSO8-1 line, PSO8-1 clone4 (e) and CD8+PSO8 line and PSO8 clone5 (g) stimulated with autologous B-LCLs pulsed with different doses of 15aa-overlapping peptides P1-to-P7 for 3 days. Percentages of BrdU+T cells (% of BrdU incorp) were determined by flow cytometry as inFig. 1. (b,d,f,h) T-cell lines and clones were cultured for 3 days with either unpulsed or 13–15aa (b,d,f) or 9–10aa (h) peptide-loaded irradiated HLA-matched B-LCLs (b,d,f) or transfectants (TX) (h) in the presence/absence of anti-HLA ClassII (aCLII) (for CD4+T-cell lines and clones) (b,d,f) or anti-HLA ClassI (aCLI) or anti-HLA-C antibodies (for CD8+T-cell lines and clones (h)). Percentage of BrdU+T cells (% of BrdU incorp) was determined by flow cytometry as inFig. 1. In all figures of panelsb,d,f,hthe three experiments mean±s.e.m. are reported. For dose–response curves in Panelsa,c,e,gwe report one representative out of three experiments performed with each T-cell line/clone. Figure 4: Epitope mapping of LL37-specific T-cell lines and clones of psoriasis patients. ( a , c , e , g ) Percentage of BrdU incorporation in psoriatic CD4 + T-cell lines PSO4-1 ( a ), PSO17-1 line, PSO17-1 clone3 ( c ), PSO8-1 line, PSO8-1 clone4 ( e ) and CD8 + PSO8 line and PSO8 clone5 ( g ) stimulated with autologous B-LCLs pulsed with different doses of 15aa-overlapping peptides P1-to-P7 for 3 days. Percentages of BrdU + T cells (% of BrdU incorp) were determined by flow cytometry as in Fig. 1 . ( b , d , f , h ) T-cell lines and clones were cultured for 3 days with either unpulsed or 13–15aa ( b , d , f ) or 9–10aa ( h ) peptide-loaded irradiated HLA-matched B-LCLs ( b , d , f ) or transfectants (TX) ( h ) in the presence/absence of anti-HLA ClassII (aCLII) (for CD4 + T-cell lines and clones) ( b , d , f ) or anti-HLA ClassI (aCLI) or anti-HLA-C antibodies (for CD8 + T-cell lines and clones ( h )). Percentage of BrdU + T cells (% of BrdU incorp) was determined by flow cytometry as in Fig. 1 . In all figures of panels b , d , f , h the three experiments mean±s.e.m. are reported. For dose–response curves in Panels a , c , e , g we report one representative out of three experiments performed with each T-cell line/clone. Full size image Similarly, the epitope specificity found in T-cell lines/clones was observed in primary proliferation assays setup from the same patients (PSO4, PSO17 and PSO8), although we observed reactivity towards additional epitopes in these assays ( Supplementary Fig. 8 ). Dose–response curves of cytokines production of T-cell lines/clones in response to LL37 and LL37 peptides are reported in Supplementary Fig. 9 . The majority of the CD4 + but not the CD8 + T-cell lines/clones produced IL-17 together with other pathogenic cytokines. CD4 + T-cell clones (PSO17 clone3, PSO8-1 clone4) co-produce IL-17 and IFN-γ, confirming the existence of T cells producing both Th1 and Th17 cytokines in psoriasis [31] . Cytokine intracellular staining of LL37-specific T-cell lines PSO4-1, PSO17-1 and PSO8-1 also confirmed the presence of IL-17/IFN-γ co-producing cells together with T cells producing only IL-17 or IFN-γ, whereas CD8 + T cell lines (PSO8, PSO41, PSO1) produced significant amounts of IFN-γ, but negligible IL-17 ( Supplementary Fig. 10 ). LL37-specific T cells show effector cell phenotype Further characterization of LL37-specific T-cell lines/clones revealed that the CD4 + T cells secreted consistent amounts of CXCL8 (also called IL-8) [32] , [33] , [34] on LL37 recognition ( Fig. 5a ). Stimulation with phorbol myristate acetate plus ionomycin (PMA+Iono), as shown for PSO17 Clone3 (to exclude contamination by accessory cells) ( Fig. 5b ), confirmed CD3 + cells being truly CXCL8 producers and in a peptide–dose-dependent manner ( Fig. 5c ). The CD8 + T-cell clone PSO8 clone5 did not produce CXCL8, but expressed perforins/granzymeB ( Fig. 5d ). Accordingly, increased perforin expression was detectable in circulating LL37-responsive CD8 + T cells ( Fig. 5e ). Following antigen stimulation, the CD8 + T-cell clone PSO8 clone5 upregulated CD107a, a marker of cytotoxic granule release [35] ( Fig. 5f ), and killed CSFE-labelled cognate targets ( Fig. 5g ). These results suggested that psoriatic LL37-specific CD4 + and CD8 + T cells, besides Th1/Th17-secretion ability, possessed direct chemotactic activity for inflammatory cells via production of CXCL8 (refs 32 , 33 , 34 ) and cytotoxic ability via perforins/granzymeB release, respectively. 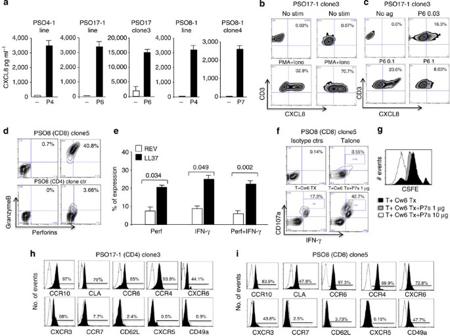Figure 5: LL37-specific T cells are effector cells producing CXCL8 and perforins/granzymeB. (a) CXCL8 measurement by the Th1/Th2 10-Plex and human IL-17 Tissue Culture Kits in the culture supernatants of T-cell lines/clones (as indicated), cultured with autologous irradiated PBMCs pulsed with no peptide (−) or 1–10 μg ml−1(depending on the T-cell line/clone) of each cognate LL37-peptide (as indicated). Results are the mean of three experiments performed with each T-cell line/clone. S.e.m. values are indicated. (b) CXCL8 staining of either unstimulated (no stim) or stimulated (PMA+Iono) CD4+T cells of PSO17 clone3 and PSO8-1 clone4; (c) CXCL8 staining of PSO17 clone3 stimulated with unpulsed(No ag)-B-LCLs or B-LCLs pulsed with the indicated doses of P6 (μg ml−1). Percent of CXCL8+CD3+cells in (b,c) is indicated on Zebra-plots derived from one of three experiments. (d) Percent of positivity for perforins/granzymeB of T-cell clones is indicated on flow cytometry contour-plots from one of three esperiments. (e) PBMCs of PSO patients responding with CD8+T-cell proliferation were cultured for 5 days with LL37 or REV. Cells were stained with anti-CD3,CD8, BrdU, perforins and IFN-γ antibodies. IFN-γ/perforins expression levels were evaluated on CD3+/CD8+cells that incorporated BrdU. Percent of expression of perforins/IFN-γ is reported compared with % of expression of the same marker in CD3+/CD8+cells stimulated with REV. Results are cumulative data derived from five independent experiments performed with different LL37-responder patients. Horizontal bars represent the mean, vertical bars are the s.e.m.Pvalues by Student’st-test for paired samples. (f) CD107a/IFN-γ staining of the CD8+T-cell clone PSO8 clone5 unstimulated (T alone) or cultured with Cw6*02+trasfectants unpulsed (T+Cw6TX) or pulsed with peptide P7s (T+Cw6TX+P7s). CD107a/IFN-γ positivity is indicated, one of three experiments is shown. (f) Flow cytometry histograms of CFSE-stained unpulsed or P7s-pulsed transfectants (as indicated) co-cultured with CD8+T-cell clone PSO8 clone5 for 6 h. One of three experiments is shown. (h,i) Markers expression on CD3+/CD4+cells (h) or CD3+/CD8+cells (i) over isotype-matched controls flow cytometry histograms. One of three to four experiments is shown for each marker. Figure 5: LL37-specific T cells are effector cells producing CXCL8 and perforins/granzymeB. ( a ) CXCL8 measurement by the Th1/Th2 10-Plex and human IL-17 Tissue Culture Kits in the culture supernatants of T-cell lines/clones (as indicated), cultured with autologous irradiated PBMCs pulsed with no peptide (−) or 1–10 μg ml −1 (depending on the T-cell line/clone) of each cognate LL37-peptide (as indicated). Results are the mean of three experiments performed with each T-cell line/clone. S.e.m. values are indicated. ( b ) CXCL8 staining of either unstimulated (no stim) or stimulated (PMA+Iono) CD4 + T cells of PSO17 clone3 and PSO8-1 clone4; ( c ) CXCL8 staining of PSO17 clone3 stimulated with unpulsed(No ag)-B-LCLs or B-LCLs pulsed with the indicated doses of P6 (μg ml −1 ). Percent of CXCL8 + CD3 + cells in ( b , c ) is indicated on Zebra-plots derived from one of three experiments. ( d ) Percent of positivity for perforins/granzymeB of T-cell clones is indicated on flow cytometry contour-plots from one of three esperiments. ( e ) PBMCs of PSO patients responding with CD8 + T-cell proliferation were cultured for 5 days with LL37 or REV. Cells were stained with anti-CD3,CD8, BrdU, perforins and IFN-γ antibodies. IFN-γ/perforins expression levels were evaluated on CD3 + /CD8 + cells that incorporated BrdU. Percent of expression of perforins/IFN-γ is reported compared with % of expression of the same marker in CD3 + /CD8 + cells stimulated with REV. Results are cumulative data derived from five independent experiments performed with different LL37-responder patients. Horizontal bars represent the mean, vertical bars are the s.e.m. P values by Student’s t -test for paired samples. ( f ) CD107a/IFN-γ staining of the CD8 + T-cell clone PSO8 clone5 unstimulated (T alone) or cultured with Cw6*02 + trasfectants unpulsed (T+Cw6TX) or pulsed with peptide P7s (T+Cw6TX+P7s). CD107a/IFN-γ positivity is indicated, one of three experiments is shown. ( f ) Flow cytometry histograms of CFSE-stained unpulsed or P7s-pulsed transfectants (as indicated) co-cultured with CD8 + T-cell clone PSO8 clone5 for 6 h. One of three experiments is shown. ( h , i ) Markers expression on CD3 + /CD4 + cells ( h ) or CD3 + /CD8 + cells ( i ) over isotype-matched controls flow cytometry histograms. One of three to four experiments is shown for each marker. Full size image We next analysed whether LL37-specific T-cell clones expressed skin-homing receptors to direct them into inflamed psoriatic skin [36] , [37] . PSO17-1 clone3 and PSO8-1 clone4 (not shown) and CD8 + T-clone PSO8 clone5 expressed all these receptors, but not the irrelevant receptors CXCR5, nor CCR7 and CD62L, lymph-node-homing receptors [38] . The CD8 + but not CD4 + T-cell clones expressed CD49a (also called VLA-1), a key molecule for trafficking of CD8 + T cells into psoriatic epidermis [39] ( Fig. 5h,i ). Thus, LL37-specific T cells seemed equipped with receptors suitable for trafficking into inflamed skin. LL37-specific T cells possess skin-homing abilities To further prove the skin-homing capability of LL37-specific T cells, we performed primary proliferation assays in which we assessed expression of skin-homing receptors in LL37-specific T cells incorporating BrdU in response to LL37 stimulation. T cells proliferating to LL37 had a higher expression of skin-homing receptors as compared with BrdU-negative T cells ( Fig. 6a ). Cumulative data in Fig. 6b show that CCR4, CCR6, CCR10 and CLA were significantly upregulated in LL37-reactive T cells. Interestingly two patients with severe disease (PSO4, PASI=18 and PSO8, PASI=20) tended to have a higher expression of skin-homing receptors, in particular CCR6 and CLA, than a patient with a mild disease (PSO17) ( Supplementary Fig. 11a ). A similar array of skin-homing receptors was expressed by T-cell lines derived from the same three patients ( Supplementary Fig. 11b ). These data indicated that circulating LL37-specific T cells harboured inflamed skin-homing receptors, a chemokine receptor array that is maintained in cultured LL37-specific T cells (at least in the T cell clones and lines analysed in this study). 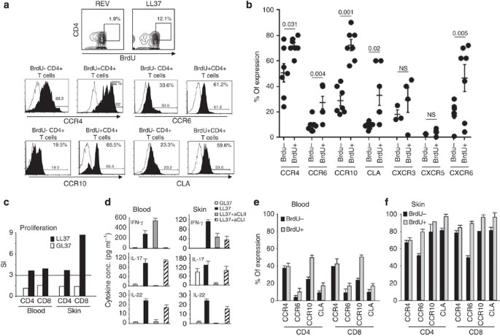Figure 6: Circulating LL37-specific T cells express skin-homing receptors and can be found in lesional psoriatic skin. (a) Representative flow cytometry countour plots (for BrdU incorporation) and histograms of expression of skin-homing receptors in primary T cells responding to LL37 (BrdU+) as compared with BrdU−T cells. One representative out of seven experiments performed with different psoriatic patients is reported. (b) Cumulative data of chemokine receptors expression in seven psoriasis patients responding to LL37 compared with the same chemokine receptor expression on BrdU−T cells.Pvalues by Student’st-test for paired samples refer to comparison between each receptor expression in BrdU−T cells and expression of the receptor in BrdU+T cells of each patient. (c) BrdU staining of patient PSO9-derived blood- and skin-T cells stimulated with autologous irradiated PBMCs pulsed with LL37 or GL37. (d) Cytokines, measured at day 2 produced by T cells stimulated as in (d), plus/minus blocking anti-HLA ClassI or -ClassII antibodies. S.e.m. values refer to triplicate cultures in the same experiment. Skin-homing receptors expression by blood (e) and skin (f) by LL37-proliferating T cells (BrdU+) and non-proliferating T cells (BrdU−) of the same experiment shown in Panelsd–f. Figure 6: Circulating LL37-specific T cells express skin-homing receptors and can be found in lesional psoriatic skin. ( a ) Representative flow cytometry countour plots (for BrdU incorporation) and histograms of expression of skin-homing receptors in primary T cells responding to LL37 (BrdU + ) as compared with BrdU − T cells. One representative out of seven experiments performed with different psoriatic patients is reported. ( b ) Cumulative data of chemokine receptors expression in seven psoriasis patients responding to LL37 compared with the same chemokine receptor expression on BrdU − T cells. P values by Student’s t -test for paired samples refer to comparison between each receptor expression in BrdU − T cells and expression of the receptor in BrdU + T cells of each patient. ( c ) BrdU staining of patient PSO9-derived blood- and skin-T cells stimulated with autologous irradiated PBMCs pulsed with LL37 or GL37. ( d ) Cytokines, measured at day 2 produced by T cells stimulated as in ( d ), plus/minus blocking anti-HLA ClassI or -ClassII antibodies. S.e.m. values refer to triplicate cultures in the same experiment. Skin-homing receptors expression by blood ( e ) and skin ( f ) by LL37-proliferating T cells (BrdU + ) and non-proliferating T cells (BrdU − ) of the same experiment shown in Panels d – f . Full size image We next took advantage of availability of skin biopsies from two psoriasis patients to test whether LL37-specific T cells could be found in lesional skin. The first patient (PSO9) had a positive response of blood T cells to LL37, whereas a second patient (PSO12) did not. LL37-specific T cells were indeed present in lesional psoriatic skin of PSO9 ( Fig. 6c ), as assessed by analysis of single-cell suspensions obtained from skin biopsies. Patient PSO9, with consistent levels of LL37-specific T cells in peripheral blood, showed detectable reactivity to LL37 of both CD4 + and CD8 + T cells from lesional skin ( Fig. 6c ). On the basis of these stimulation indexes, CD8 + T cells proliferated more in the skin than in blood in this patient. Both CD4 + and CD8 + skin-derived T cells produced IFN-γ, but only CD4 + T cells produced Th17 cytokines ( Fig. 6d ), confirming observations made with LL37-specific T cells in blood of other psoriasis patients (see above). LL37-specific skin T cells, gated as BrdU + T cells, expressed the highest amounts of CCR10, CLA and CCR6 ( Fig. 6e,f ). Thus, in both blood ( Fig. 6e ) and skin ( Fig. 6f ), T cells proliferating to LL37 showed an increased percentage of expression of skin-homing receptors. Altogether, these results indicated that LL37-specific T cells had ability to migrate into psoriatic skin lesions and that these T cells can proliferate and produce pathogenic cytokines when stimulated in vitro with LL37. Blood LL37-specific T cells are visualized by HLA tetramers To definitely prove that LL37 is an autoantigen in psoriasis, we produced HLA-ClassII/I tetramers expressing the peptides recognized by some T-cell lines/clones described above (see Methods). CD4 + PSO17-1 line and clone3, specific for P6, could be stained with a DR11 tetramer harbouring this peptide (DR11-P6-tetramer) but not an irrelevant tetramer loaded with peptides P4 (DR11-P4 tetramer) (indeed, P4 did not stimulate these T cells) ( Fig. 7a ). Instead, line PSO4-1, specific for P4 and not P6, stained positive with the DR11-P4, but not DR11-P6 tetramer (P6 was not recognized by line PSO4) ( Fig. 7b ). Tetramers of Cw6*02 molecules loaded with short peptides P6s and P7s, (Cw6*02-P6s and -P7s tetramers) stained the CD8 + T-cell line PSO8 and PSO8 clone5 ( Fig. 7c,d ). As expected, the P7s-Cw6*02 tetramer yielded stronger staining as compared with the P6s-Cw6*02-tetramer, in that peptide P7s was a stronger agonist than peptide P6s for LL37-specific CD8 + T cells of patient PSO8. 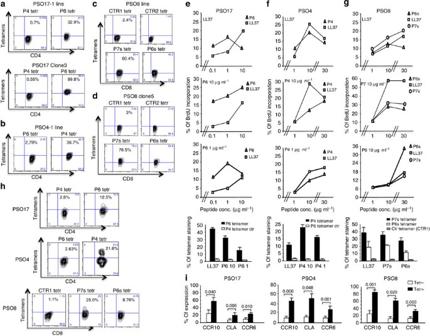Figure 7: LL37-specific T cells are identified by tetramer staining. (a–d) PSO17-1, PSO17 clone3 (a) and PSO4-1 (b) CD4+T cells were stained with cognate-tetramer DR11-P6 (P6 tetr) or control DR11-P4 (P4 tetr) (a) or cognate DR11-P4 or control DR11-P6 tetramer (b) followed by CD4 staining and 7ADD labelling to exclude dead cells; CD8+T cells of patient PSO8 (T cell line PSO8,c) and PSO8 clone5 (d) were stained with Cw6*02-P6s or Cw6*02-P7s tetramers (P6s tetr or P7s tetr) or control tetramers B27*05-LMP (CTR1 tetr) or HLA-A2-CMV (CTR2 tetr) followed by CD8 staining and 7ADD labelling. Flow cytometry contour plots from one out of three to four experiments performed with each T-cell line/clone. (e–g) PBMCs of patients PSO17 (e), PSO4 (f), PSO8 (g) were cultured for 6 days with LL37 (LL37) or LL37 peptides as indicated, washed and stimulated with irradiated autologous PBMCs pulsed with LL37/LL37-peptides (as indicated; proliferation assessed as inFig. 1). Each bulk culture was stained with cognate tetramers (DR11-P6 tetramer for PSO17 bulk-cultures, DR11-P4 tetramer for PSO4 bulk cultures and Cw6*02-P7s and Cw6*02-P6s tetramers for PSO8 bulk cultures) and control tetramers (DR11-P4 for PSO17 bulk cultures, DR11-P6 for PSO4 bulk cultures and B27*05 LMP for PSO8 bulk cultures) as in (a–d); percentages of tetramer staining are reported as histogram graphs ±s.e.m. of triplicate cultures (lower graphs ofe–g). (h) Blood T cells of PSO17, PSO4 (CD3+CD4+) and PSO8 (CD3+CD8+) patients were cultured for 2 days with LL37, stained with the same cognate and control tetramers as in panelsa–dande–g, followed by staining with anti-CD3/CD38 antibodies; tetramer staining was analysed by flow cytometry on CD3+CD4+CD38highor CD3+CD8+CD38highcells. Flow cytometry contour plots from one out of three experiments performed with each patient. (i) T cells stained with tetramers (tetr+) or T cells negative for tetramer staining (tetr-) of PSO17, PSO4 and PSO8 patients were analysed for CCR10, CCR6 and CLA expression, by flow cytometry. Percent of expression of each marker is shown as histograms representing the mean of three experiments (±s.e.m.) performed with each patient for each marker.Pvalues by Student’st-test for paired samples. Figure 7: LL37-specific T cells are identified by tetramer staining. ( a – d ) PSO17-1, PSO17 clone3 ( a ) and PSO4-1 ( b ) CD4 + T cells were stained with cognate-tetramer DR11-P6 (P6 tetr) or control DR11-P4 (P4 tetr) ( a ) or cognate DR11-P4 or control DR11-P6 tetramer ( b ) followed by CD4 staining and 7ADD labelling to exclude dead cells; CD8 + T cells of patient PSO8 (T cell line PSO8, c ) and PSO8 clone5 ( d ) were stained with Cw6*02-P6s or Cw6*02-P7s tetramers (P6s tetr or P7s tetr) or control tetramers B27*05-LMP (CTR1 tetr) or HLA-A2-CMV (CTR2 tetr) followed by CD8 staining and 7ADD labelling. Flow cytometry contour plots from one out of three to four experiments performed with each T-cell line/clone. ( e – g ) PBMCs of patients PSO17 ( e ), PSO4 ( f ), PSO8 ( g ) were cultured for 6 days with LL37 (LL37) or LL37 peptides as indicated, washed and stimulated with irradiated autologous PBMCs pulsed with LL37/LL37-peptides (as indicated; proliferation assessed as in Fig. 1 ). Each bulk culture was stained with cognate tetramers (DR11-P6 tetramer for PSO17 bulk-cultures, DR11-P4 tetramer for PSO4 bulk cultures and Cw6*02-P7s and Cw6*02-P6s tetramers for PSO8 bulk cultures) and control tetramers (DR11-P4 for PSO17 bulk cultures, DR11-P6 for PSO4 bulk cultures and B27*05 LMP for PSO8 bulk cultures) as in ( a – d ); percentages of tetramer staining are reported as histogram graphs ±s.e.m. of triplicate cultures (lower graphs of e – g ). ( h ) Blood T cells of PSO17, PSO4 (CD3 + CD4 + ) and PSO8 (CD3 + CD8 + ) patients were cultured for 2 days with LL37, stained with the same cognate and control tetramers as in panels a – d and e – g , followed by staining with anti-CD3/CD38 antibodies; tetramer staining was analysed by flow cytometry on CD3 + CD4 + CD38 high or CD3 + CD8 + CD38 high cells. Flow cytometry contour plots from one out of three experiments performed with each patient. ( i ) T cells stained with tetramers (tetr+) or T cells negative for tetramer staining (tetr-) of PSO17, PSO4 and PSO8 patients were analysed for CCR10, CCR6 and CLA expression, by flow cytometry. Percent of expression of each marker is shown as histograms representing the mean of three experiments (±s.e.m.) performed with each patient for each marker. P values by Student’s t -test for paired samples. Full size image Repetitive stimulations with LL37 may induce an in vitro priming/expansion of T cells that are not present in vivo . To exclude this, we made primary bulk cultures by using either LL37 or LL37 peptides as stimulators. After a 6-day culture we performed criss-cross experiments to check specificity. Not only the bulk culture T cells obtained in the first place with LL37 recognized once again peptides P6 (PSO17, Fig. 7e ), P4 (PSO4, Fig. 7f ) and P6s/P7s (PSO8, Fig. 7g ), vice versa, T cell expanded with LL37 peptides recognized full-length LL37. This suggested that LL37 and LL37 peptides expanded comparable T-cell repertoires and peptide-antigens discovered by epitope mapping were indeed physiologically generated on LL37 processing. Percent of staining with tetramers loaded with the cognate peptide paralleled antigen reactivity to the same peptide, as determined by BrdU assay ( Fig. 7e,g , lowest panels). Altogether, these data suggest that LL37 tetramers were very sensitive in discriminating subtle differences in T-cell reactivity of LL37-specific T-cell lines and clones, suggesting that they could be used to track LL37-specific T cells in blood of psoriatic patients. Tetramer labelling was assessed on activated T cells [40] after a 48-hour culture of PBMCs with LL37. A clear determination of tetramer-positive T cells was evident in the three patients analysed in Fig. 7h . Tetramer-positive T cells also showed increased percentage of staining for skin-homing receptors CCR10, CLA and CCR6 compared with BrdU − T cells ( Fig. 7i ). Healthy donors that were LL37 unresponsive, matched for HLA-DR11 or Cw6*02 expression with patients PSO4 and PSO17 or PSO8, respectively, did not show any positive staining with the same tetramers ( Supplementary Fig. 12 ). These experiments allowed the definitive identification of LL37-specific T cells in psoriasis patients. LL37-specific T cells change after disease remission Finally, we asked how LL37-specific T cells behave during the treatment course of psoriasis. We monitored PASI scores and LL37-specific T-cell responses in two patients receiving anti-TNF-α therapy. Patients PSO4 and PSO8 started with PASI 18 and 20, respectively, and reached PASI75 (a reduction of 75% of the initial PASI score) after treatment ( Fig. 8a ). Paralleling disease amelioration we observed a significant reduction in circulating LL37-specific T cells detected by BrdU incorporation ( Fig. 8b ) and lower tetramer staining ( Fig. 8c ). Interestingly, circulating LL37-specific T cells also showed marked reduction of skin-homing receptors CCR10, CLA, CCR6 ( Fig. 8d–f ). Ameliorating patients PSO4 and PSO8 produced low IFN-γ in response to LL37 ( Fig. 8g,h ). LL37-specific T cells of patient PSO4, produced high levels of IL-17 at the time of PASI 18, so that IL-17 release was easily detected by ELISA in culture supernatants collected during primary proliferation assays. Such T cells also produced a discrete amount of IL-22. After disease improvement LL37-specific T cells of PSO4 lost ability to produce IL-17 and produced less IL-22 ( Fig. 8g,h ). LL37-specific T cells of patient PSO8, besides reducing IFN-γ production in response to LL37, acquired IL-10 secretion ability ( Fig. 8g,h ). These results showed that clinical psoriasis course is paralleled by quantitative and qualitative changes in circulating LL37-specific T cells. We also analysed patient PSO17 with mild psoriasis (PASI 5) that did not change significantly over time. Compared with PSO4 and PSO8, LL37-specific T cells from PSO17 were less frequent, expressed lower levels of skin-homing receptors CCR10, CLA, CCR6 and displayed lower cytokine secretion capacity. Altogether, these data suggested that phenotype and intensity of peripheral LL37-specific T-cell responses correlated with disease activity. 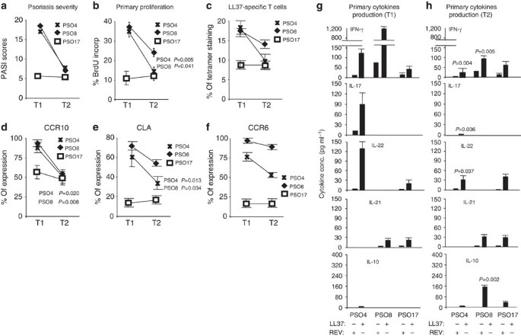Figure 8: LL37-specific T-cell responses persist during disease amelioration, but change in intensity and quality. (a) Time-dependent evolution of psoriasis severity (PASI) in patients PSO4, PSO8 and PSO17. (b) Time-dependent primary T-cell proliferation to LL37, (c) tetramer staining performed as reported inFig. 6h, (d) CCR10, (e) CLA and (f) CCR6 staining (measured as inFigs 4 and 5) of PBMCs of patients PSO4, PSO8, PSO17. Proliferation is given as percent of BrdU incorporation by T cells in response to LL37 minus proliferation to control peptide. Data of tetramer detection in blood T cells are reported as percent of tetramer staining with cognate tetramers (tetramer DR11-P4 for patient PSO4, tetramer DR11-P6 for patient PSO17 and tetramer Cw6*02-Ps7 for patient PSO8) minus binding of the control irrelevant tetramer (DR11-P6 tetramer for patient PSO4, DR11-P4 tetramer for patient PSO17 and B27*05-LMP (CTR1) tetramer for patient PSO8). Data are the mean of three experiments (% of expression of BrdU or CCR10, CLA, CCR6 receptors or tetramers in CD3+cells from each patient at each time point) and are reported in the graph ±s.e.m.Pvalues by Student’st-test for paired samples are indicated. (g,h) Measurement of cytokine secretion in culture supernatants of PBMCs stimulated at T1(g) and T2(h) with LL37 or REV peptide (as indicated) for 3 days in the same patients as in (a–f). Results are reported as cytokine concentrations measured by ELISA. Data are the mean of three experiments and are reported as histograms ±s.e.m.Pvalues by Student’st-test for paired samples refer to decrease (for IFN-γ, IL-17, IL-22) or increase (IL-10) of each cytokine detected by ELISA in primary proliferation assays at T2 with respect to the production of the same cytokine at T1. Figure 8: LL37-specific T-cell responses persist during disease amelioration, but change in intensity and quality. ( a ) Time-dependent evolution of psoriasis severity (PASI) in patients PSO4, PSO8 and PSO17. ( b ) Time-dependent primary T-cell proliferation to LL37, ( c ) tetramer staining performed as reported in Fig. 6h , ( d ) CCR10, ( e ) CLA and ( f ) CCR6 staining (measured as in Figs 4 and 5 ) of PBMCs of patients PSO4, PSO8, PSO17. Proliferation is given as percent of BrdU incorporation by T cells in response to LL37 minus proliferation to control peptide. Data of tetramer detection in blood T cells are reported as percent of tetramer staining with cognate tetramers (tetramer DR11-P4 for patient PSO4, tetramer DR11-P6 for patient PSO17 and tetramer Cw6*02-Ps7 for patient PSO8) minus binding of the control irrelevant tetramer (DR11-P6 tetramer for patient PSO4, DR11-P4 tetramer for patient PSO17 and B27*05-LMP (CTR1) tetramer for patient PSO8). Data are the mean of three experiments (% of expression of BrdU or CCR10, CLA, CCR6 receptors or tetramers in CD3 + cells from each patient at each time point) and are reported in the graph ±s.e.m. P values by Student’s t -test for paired samples are indicated. ( g , h ) Measurement of cytokine secretion in culture supernatants of PBMCs stimulated at T 1 ( g ) and T 2 ( h ) with LL37 or REV peptide (as indicated) for 3 days in the same patients as in ( a – f ). Results are reported as cytokine concentrations measured by ELISA. Data are the mean of three experiments and are reported as histograms ±s.e.m. P values by Student’s t -test for paired samples refer to decrease (for IFN-γ, IL-17, IL-22) or increase (IL-10) of each cytokine detected by ELISA in primary proliferation assays at T2 with respect to the production of the same cytokine at T1. Full size image Psoriasis has long been considered a T-cell-mediated autoimmune disease [41] , although the nature of the autoantigen/s recognized by the pathogenic T cells remained poorly understood. Keratinocyte-derived proteins [18] , [19] , [20] , [21] , [22] , [42] , among which keratins, were previously identified as autoantigens, especially in a subset of patients with psoriasis linked to group-A β-hemolytic streptococcal throat infections. Our study now identifies the AMP LL37 as a new autoantigen in psoriasis that is recognized by circulating T cells in 46% of psoriasis patients and up to 75% of patients with moderate-to-severe psoriasis. By studying a subgroup of psoriasis patients, we also found that 26 and 8.7% of patients harboured circulating T cells that respond to Keratin17 and Keratin6, respectively. Responses to Keratin17 were present in patients with more severe diseases (not shown) and were statistically significant, which is in keeping with literature suggesting that Keratin17 is the most immunogenic among keratins [22] . Reactivity to keratins is explained by ‘molecular mimicry’ phenomena due to sequence homologies between keratins and streptococcal protein M [21] . For an AMP such as LL37 autoreactivity is unlikely the result of ‘molecular mimicry’ but it could be rather the consequence of intrinsic properties of LL37. Indeed, the continuous overexpression of LL37, which may be linked to the genetic background, coupled with sustained LL37-mediated TLR activation of DCs on formation of LL37 extracellular self-nucleic acids complexes [13] , [14] may drive the break of T-cell tolerance to LL37. Many studies have pointed out a key role of conventional DCs in this process, although participation of pDCs, shown to prime IL-22-producing T cells with skin-homing capacity, cannot be excluded [43] . In this scenario, LL37 represents the first example of an AMP that, besides acting as an adjuvant [13] , [14] , [15] for innate immune cell activation, is recognized as an autoantigen by T cells in autoimmune settings. LL37-specific T cells belong to both CD4 + and CD8 + T-cell compartments, consistent with their role in psoriasis pathogenesis. Accordingly, HLA-binding predictions suggest that LL37-derived fragments potentially bind to several HLA-DR and ClassI alleles. Our binding assays to the most common HLA-DR alleles DR1, DR4, DR11 further suggest the presence of ‘promiscuous HLA-DR-binding epitopes’ within LL37 sequence. Also, epitope preference for peptides P1, P4, P6, P7 concords with prediction analyses performed with MHC-binding prediction servers: these sequences possess the highest scores for binding to HLA-alleles DR1, DR4, DR11 as well as DR7 and DR16. A discrete number of LL37 fragments are Cw6*02 binders and accordingly we found LL37-specific responses restricted to CD8 T cells by Cw6*02. Among 11 patients with LL37-specific CD8 + T cells, five were Cw6*02 + and this is approximately the expected frequency of Cw6*02 in psoriasis-affected individuals [26] , [27] , [28] . Although the data are not sufficient at present to indicate a particular ability of Cw6*02 to serve as restriction element for LL37-presentation as compared with other HLA-ClassI alleles, the data suggest that other HLA-ClassI alleles may also act as restriction elements. The possibility of ‘promiscuous’ HLA-binding abilities of LL37-derived peptides can explain why LL37 reactivity is frequently detected in psoriasis, independently of patient’s HLA background. We have not HLA-DR typed all patients included in the present study; thus, we do not know whether the distribution of the most common HLA-DR alleles is altered in psoriasis patients responding to LL37. At present while the association of ClassI-Cw6*02 allele with type I psoriasis is well established [26] , [27] , [28] , the association with HLA-DR alleles is not completely clear. Some studies are in agreement with the fact that some HLA-ClassII alleles are more commonly found in association with the Cw6*02 allele, as it is the case for HLA-DR7 (HLA-DRB1*07) [44] . Of note, one patient in our study (PSO8) responded to LL37 by presenting CD8-restricted epitopes via Cw6*02 and CD4-restricted epitopes via HLA-DR7. Whether other AMPs overexpressed in psoriatic skin are autoantigens is under investigation. In our hands HBD2, overexpressed in psoriasis and capable of pDC activation by complexing with nucleic acids [45] , was unable to stimulate psoriatic T cells. According to prediction analysis for HLA-DR binding, HBD2 sequence results less promiscuous than LL37, but this may not be sufficient to explain lack of immunogenicity. LL37-specific T cells produced IFN-γ and Th17 cytokines in both blood and skin. Such cytokines exert well-known pathogenic effects in skin lesions [4] , [5] , [6] , [7] , [8] , [9] , [31] . Interestingly, LL37-specific T cells of a patient with rare exacerbation episodes and a patient improving symptoms produced IL-10 and low IFN-γ. In another remitting patient LL37-specific T cells lost IL-17-secretion capacity. Noteworthy, the two improving patients received Etanercept, a TNF-α blocker reported to inhibit IL-17 and increase IL-10 production by T cells [46] , [47] . Emergence of IL-10 plus vanishing of IFN-γ/Th17 responses in patients that lowered PASI is consistent with the correlation that we found between presence of LL37-specific T cells producing IFN-γ, IL-17, IL-21, IL-22 (refs 7 , 8 , 9 , but not Tregs/Th2-cytokines IL-10/IL-4) with moderate-to-severe psoriasis. Results confirmed at clonal level also suggest additional pro-inflammatory potential of LL37-specific CD4 + T cells via consistent CXCL8 secretion. Like pathogenic T cells reported in other chronic disorders CXCL8-producing T cells expressed CCR6 and may drive neutrophil recruitment [32] , [33] , [34] . In our assays, blood LL37-specific CD8 + T cells were less frequently detected than CD4 + T cells. However, some T cells (especially CD8 + ) are segregated from the circulating lymphocyte pool as ‘tissue-resident memory cells’ (T RM ) [48] . Likely, LL37-specific CD8 + T cells accumulate in the skin as T RM where they exert pathogenic effects via IFN-γ secretion. As an alternative explanation CD8 + T cells in blood of psoriasis patients could be effector cells with poor proliferative capacity. Although CD8 + T cells may be the ultimate effectors in psoriatic skin inflammation, CD4 + T cells are also crucial in psoriasis. Indeed, the CD4 + T cells, like the CD8 + T cells, show oligoclonal expansion in psoriatic skin [49] , [50] . Activated CD4 + T cells have been shown to induce a psoriasiform inflammation in epidermal cells in a recently set up 3D model of inflammatory skin disease [51] . In the past, it has been shown that injection of pre-psoriatic skin with CD4 + , and not CD8 + T cells, induced psoriasis [52] . This phenomenon induces the recruitment of other T cells among which are high amounts of CD8 + T cells [52] . As CD4 + T cells are crucial for inducing cross-priming of CD8 + T cells [53] and maintenance of their effector functions, the activation of autoreactive LL37-specific CD4 + T cells in psoriasis may sustain effector functions of CD8 + T cells specific for LL37 itself and/or other autoantigens (included Keratins). Although recent literature showed that CD8 + T cells produce Th17 cytokines in psoriasis [54] , this was not confirmed in our study, however we cannot exclude the existence of CD8 + T cells with such characteristics in other patients. The role of T-cell-derived IFN-γ in psoriasis, a disease with an IFN-γ-genomic signature [55] , should not be underscored. IFN-γ activates keratinocytes, induces inflammatory chemokines/cytokines [31] , [56] , [57] , [58] and produces histological features of psoriatic lesions when injected in non-lesional psoriasis skin [59] . Indeed, a recent mouse model of psoriatic skin inflammation showed CD8 + T cells being critical players via IFN-γ secretion [60] . LL37-specific CD8 + T cells have some features of cytotoxic effector cells in line with perforins/granzymesB being found in psoriasis lesions [61] . However, it is difficult to reconcile the role of T-cell-mediated cytotoxicity with the reported resistance of psoriatic keratinocytes to killing [62] (for review see ref. 61 ). Altogether, features of LL37-specific T cells described here support their role as pathogenic actors in psoriasis, corroborated by their skin-homing ability. We have not performed systematic analyses in all patients of chemokine receptor expression that would correlate with psoriasis activity. However, LL37-specific T cells of patients with moderate-to-severe disease mostly expressed higher amounts of skin-specific CCR10, CLA and CCR6 as assessed in primary proliferation assays. Moreover, these receptors decreased in LL37-specific T cells on clinical remission. Increased CLA expression by T cells was described in severe psoriasis [63] . Interestingly, it has been shown that IL-4 down-regulates CLA [64] and we have found that LL37-specific T cells of a mild-psoriasis patient (PSO17) produce IL-4 and, accordingly, expressed lower level of CLA. In conclusion, our study demonstrates that LL37, an AMP over-expressed in psoriatic skin, represents a T-cell autoantigen in psoriasis. As LL37 is able to activate innate immune cells and break innate tolerance to self-nucleic acids [13] , [14] , [15] , it represents an even more appealing target to treat psoriasis. Therapeutic targeting of LL37-specific T cells may provide new avenues to prevent or treat psoriasis without inducing indiscriminate immunosuppression [65] . Collection of human samples This study was approved by the Institutional Review Boards of Universities Tor Vergata and La Sapienza, Rome, IT, University Hospital of Zurich, Lausanne (CHUV), CH, and MD Anderson Cancer Center (TX). Informed consent was obtained from all patients. Twenty millilitres of blood was drawn from patients with chronic plaque psoriasis, diagnosed according to standard clinical/histopathological criteria. Control blood was taken from scleroderma patients diagnosed with classification criteria by the American College of Rheumatology (ACR), healthy controls, atopic dermatitis-, and erysipelas patients, diagnosed according to standard clinical criteria. No systemic medications were administered for 8 weeks before analysis. A group of patients, receiving anti-TNF-α therapies, was also enrolled to check LL37-specific responses before and after therapy. Psoriasis plaque specimens were taken by 6-mm-punch biopsies at University of Tor Vergata, Rome. Antigens LL37, GL37, β-defensin2 (HBD2) were from Innovagen, REV from AnaSpec, LL37 peptides and matched short REV peptides by Anawa, Trading SA (Zurich, CH). Keratin6 and Keratin17 from Abnova; HNP 1-3 from Hycult Biotechnology (Canton, MA); Tetanus Toxoid (TT) from Enzo Life Science (Lausen, Switzerland). Peptide antigens used were listed in Supplementary Table 2 . ‘MHC-binding-prediction-servers’ for searching ‘HLA-binding motifs’ within LL37, HNP-1-3 and HBD2 sequences were http://www.imtech.res.in/raghava/propred/ , http://tools.immuneepitope.org/mhcii/ , http://tools.immuneepitope.org/mhci/ [23] , [24] . T-cell proliferation assay PBMCs, purified on Ficoll-Hypaque (Pharmacia Fine Chemicals, Uppsala, Sweden) were incubated (10 5 cells/well) in 96-well-flat-bottom microplates (BD) in T-cell medium (RPMI 1640, 10% heat-inactivated Human Serum (FCS, Gibco), 2 mM L -glutamine, 10 U ml −1 penicillin and 100 μg ml −1 streptomycin), with/without peptides. At day3 and 5, BrdU was added (3 μg ml −1 ). BrdU incorporation was detected by allophycocyanin(APC)-labelled anti-BrdU antibody (BD Pharmingen), after surface staining by flow cytometry. Generation/characterization of T-cell lines/clones As previously described [66] , psoriatic PBMCs were stimulated (2 × 10 6 cells ml −1 ) with LL37 for 7 days and re-stimulated (10 days) with LL37-pulsed (10 μg ml −1 ) autologous-γ-irradiated-(30Gy)-PBMCs in T-cell medium in the presence of human/recombinant(hr)IL-2 (Boehringer-Mannheim, Indianapolis, Indian, USA). T-cell line-specificity was analysed by using peptide-pulsed (10 μg ml −1 ) autologous-irradiated PBMCs or transfectants (30Greys) or lymphoblastoid-cell lines (B-LCLs) (150Greys). BrdU was added at day 2. At day 4, T cells were analysed by flow cytometry. Before cloning, bulk cultures were stimulated with autologous-irradiated PBMCs and peptide, overnight, stained with the ‘Cytokine secretion assays kits’ (MACS, Miltenyi) and anti-surface molecules (anti-CD3, anti-CD4 and/or anti-CD8 antibodies, see below in ‘Antibodies and reagents for flow cytometric analysis’) to detect IL-2, IFN-γ and/or IL-17 secretions and upregulation of activation markers (CD71, CD38) and sorted by a cell-sorter (MoFlo Astrios, Beckman Coulter). Dead cells were excluded by DAPI staining. Sorted activated CD4 + or CD8 + CD3 + cells, secreting cytokines, were cloned by limiting dilution in Terasaki plates (Nunc Microwell, Sigma-Aldrich) in the presence of allogenic-irradiated (10 4 ) PBMCs activated by phytohaemagglutinin (1 μg ml −1 , PHA, Murex, 0.5 cells per well). 100 U ml −1 −150 U ml −1 of hrIL-2 were added. Expanded clones reactivity and HLA restriction were analysed using HLA-matched-homozygous B-LCLs or HLA-transfectants (see below) pulsed with peptide antigen or control peptide antigens. Isolation/characterization of T cells from lesional skin Biopsies as described [9] were incubated overnight with 2 U ml −1 DispaseII (Roche) in PBS at 4 °C. Dermis was separated from epidermis by peeling-off epidermal sheet and cutting into small pieces, transferred into 24-well-plates in T-cell medium and rhIL-2 (100 U ml −1 ) at 37 °C. T cells, migrated from dermis after 3–4 days, were resuspended in T-cell medium and plated into 96-well-plates (2 × 10 4 cells per well) with 10 5 irradiated autologous PBMCs pulsed with LL37 and/or GL37 (10–30 μg ml −1 ) or LL37 peptides and control peptides. BrdU was added at day 1 and proliferation tested by BrdU assay at day 3. Immunohistochemistry Immunohistochemical staining was performed on 6-mm paraffined sections of human psoriasis skin specimens. Specimens were stained with a rabbit anti-LL37 (Innovagen, dilution 1:1,200) or isotype control followed by a secondary antibody anti-rabbit IgG (Vector Laboratories). HRP and DAB (DAKO) were used to develop the colour. Nuclear staining was performed with Mayer’s haematoxylin. Antibodies and reagents for flow cytometric analysis Blocking mouse-anti-human HLA-DR antibody (L243) was from BD Pharmingen (San Diego, CA) (used at 10 μg ml −1 ). Blocking mouse-anti-human HLA-ClassI (W6/32) and anti-HLA-C were from Abcam (both used at 10 μg ml −1 ). Antibodies to CD4 (OKT4), CD8 (OKT8), CD3 (OKT3), conjugated with various fluorochromes (FITC, phycoerythrin (PE), peridinin-chlorophyll-protein (PerCp), APC, PE-Cy7) were from BD Biosciences or eBiosciences (San Diego, CA). For further LL37-specific T-cell characterization, FITC-, APC-, PE-, PerCp-, PerCpCy5.5-, APC-anti-Cy7-, AlexaFluor488-conjugated anti-CCR4 (1G1), -CCR10 (314305), -CCR6 (11A9), -CLA (HECA-452), -CXCR5 (51505), -CXCR3 (1C6) -CD62L (DREG-56), -CCR7 (150503), -CXCR6 (TG3), -CD38 (HIT2), -CD71 (CY1G4) and -CD49a (TS2/7) antibodies were purchased from BD Biosciences or eBiosciences, Novus Biologicals (Littleton, CO), R&D (Minneapolis, MN), Invitrogen Life Technologies and Biologend (San Diego, CA). FITC, APC, PE, PerCp-conjugated anti-human-IFN-γ (4S.B3), -IL-17 (eBio64DEC17), -IL-22 (142928), -IL-21 (3A3-N2), -IL-4 (8D4-8), -IL-13 (JES10-5A2), -IL-5 (JES1-39D10), -IL-10 (JES3-19F1) -CXCL8 (G265-8) were from BD Pharmingen, eBiosciences, BioLegend or R&D Systems, as well as appropriate isotype-matched controls. FITC-Anti-human CD107a (eBioH4A3) and isotype matched-control were from e-Bioscence. Anti-perforins (δG9), -granzymesB antibodies (GB11), FITC-CFSE (used at 0.5 μg ml −1 ) were from BD Bioscience, PerCp-7-AAD from BD Pharmingen, DAPI from Invitrogen. Cytokine measurement in T cells Cytokine secretion was detected by enzyme-linked-immunosorbent-assay (ELISA; Quantikine; R&D Systems, Minneapolis, MN) for IL-4, IL-10, IL-17, IFN-γ, IL-22, IL-21, IL-8, IL-13, IL-1β, TNF-α or by Th1/Th2 10-Plex and IL-17-Tissue Culture Kits (read by MSD Sector Imager 2400, Meso Scale Discovery, Gaithersburg, MD). Supernatants were harvested from primary cultures at day3 (day2 for lines/clones). Production of cytokines was also analysed by flow cytometry after culture of PBMCs with LL37/LL37-peptides for 6-7 days. T cells were activated with phorbol myristate acetate (Sigma)/ionomycin (Calbiochem) (PMA+Iono) for 4 h and secretion blocked with GolgiStop (BD Biosciences). T-cell clones were cultured with HLA-matched-B-LCLs/transfectants either unpulsed/pulsed with cognate peptide-antigen overnight. Cells were permeabilized/fixed by the fixation kit eBiosciences. T cells were gated on CD3,CD4 or CD8 expression and cytokine staining analysed on BrdU + cells. Enrichment of perforins + /GranzymeB + T cells was analysed in the same way. In some experiments perforins/granzymeB were analysed after a 4-day culture with antigens on CD3 + CD4 + CD38 + or CD3 + CD8 + CD71 + cells. CD107a assay/cytotoxic assay T cells were cultured for 5 h with B-LCLs/transfectants pulsed/unpulsed with cognate antigen in continous presence of anti-CD107a or isotype-control antibody [35] . Cells were washed and stained for surface markers and/or IFN-γ as described above. To assess killing of target cells by T-cell clones, T cells were cultured with HLA-matched CFSE-labelled tranfectant pulsed/unpulsed with peptide for 6–12 h. For CFSE labelling, target cells were stained in CFSE/RPMI (10 7 cells ml −1 ) for 10 min at 37 °C and reaction was stopped with RPMI 25% FCS in ice. Residual presence of CFSE-labelled targets in culture after culture with CD8 + T cells was evaluated by flow cytometry. Peptide-competition assays For each peptide, eight wells of a v-bottom 96-well plate were filled with 50 μl of recombinant ‘empty’ HLA-DR proteins (1 μg) in citrate-saline buffer (100 mM citrate pH 6.0), 0.2% β-octyl-glucopyranoside, 1 × complete protease inhibitors, 2 μM biotin-HA306-318. Each of LL37 peptides used as competitors were added to each well to final 100, 30, 10, 3, 1, 0.3, 0.1 μM at 37 °C overnight and then each reaction was diluted with a fourfold volume of 1PBS, pH 7.4, 0.1% BSA, 0.05% Tween 20 (PBT), 100 μl applied to an anti-HLA-DR-coated plate (L243, 2 μg ml −1 ), previously blocked with PBT. After 1-hour incubation at RT and three washes with 1 × PBS pH 7.4, 0.05% Tween20, streptavidin-alkaline phosphatase (SA-AP) conjugate was added as 1:10,000 in PBT. After 1 h, the plate was washed and developed with pNPP SigmaFAST substrate and absorbance read with a 405 nm filter. Binding assay of LL37 peptides to Cw6*02 molecules Binding of LL37 peptides to Cw6*02 molecules was assessed at TC Metrix, Epalinges, CH, by ‘Small scale refolding’ (10 ml) and elution of recombinant Cw6*02 molecules in the presence of 9- to 10-aa-long LL37 peptides (ps4a, ps4b, ps5, ps6 and ps7), chosen for the presence of ‘binding motifs’ for Cw6*02 according to prediction servers (see above). Cw6*02 molecules were eluted by gel filtration (Superdex 75). Refolding of the same molecule in the presence of a non binder (negative ctr) and a good binder (positive ctr) peptide was also performed. Good binder peptides were those inducing the best re-folding of Cw6*02 molecules: this allows to detect a clear peack of elution by gel filtration. Isolation and stimulation of blood pDCs For isolation of human peripheral blood pDCs, blood buffy coats of healthy donors were obtained from the Service Regional Vaudois de Transfusion Sanguine, Lausanne, CH, and from Gulf Coast regional Blood Center, Houston, Texas. After separation of mononuclear cells by Ficoll centrifugation, pDCs were purified as described [13] by using Plasmacytoid Dendritic Cell Isolation Kit II (Miltenyi Biotec) to obtain 99% purity. Purified pDCs were seeded into 96-well round-bottom plates at 5 × 10 4 cells per well in 200 μl RPMI 1640 (GIBCO) supplemented with 10% FCS (Atlanta biologicals). LL37 and control peptides were premixed with total human genomic DNA (3 μg ml −1 ). After 30-min incubation at room temperature the mix was added to the pDC cultures. IFN-α in supernatants was measured by ELISA (PBL Biomedical Laboratories, New Brunswick, NJ) after 24 h. B-LCLs and transfectants (Tx) Cw6*02 restriction was analysed using the human B-cell line 721.221 deficient in cell surface expression of ClassI MHC proteins transfected with cDNA encoding for Cw6*02 (ref. 67 ). Other transfectants used were (1) T2 cell line, a human lymphoblastoid HLA-A2 + cell line commercially available at ATCC (TX-HLA-A2); (2) T2.DR4 (TX-DR4) generated through transfection of HLA-DRB1*0401 cDNA into T2 cells (the T2.DR4 cell line is HLA-DM deficient, making cell surface DRB1*0401 molecules receptive to loading by exogenous peptides); (3) C1R.A2 B-cell line transfected with human HLA-A1 (TX-HLA-A1) [68] . The C1R.A2 cells are negative for other HLA classI A and B alleles [67] . They were shown to be NK susceptible, which is a sensitive functional read out of HLA-ClassI deficiency, included HLA-C [69] . B-LCLs from PSO patients or HD were generated by incubating 5 × 10 5 -10 6 PBMCs with Epstein-Barr virus (EBV) from Marmoset lymphoblastoid-cell line B95-8 (ref. 66 ). B-LCLs were cultured in T25 flasks (Corning Incorporated, Corning, NY) in RPMI1640, 10% heat-inactivated Fetal Calf Serum, 2 mM L-glutamine, 10 U ml −1 penicillin and 100 μg ml −1 streptomycin (B-cellmedium), and regularly passaged. Tetramer staining of T-cell lines/clones and blood T cells LL37 tetramers used were DR11-P6 peptide, DR11-P4, Cw6*02-P6s, Cw6*02-P7s, B27*05-LMP236-244, HLA-A2-CMV-pp65, all from TC Metrix, Epalinges, CH. Staining was performed at 37 °C for 40 min for the HLA-DR tetramers and 1 h at room temperature for ClassI tetramers, followed by staining for CD4 or CD8 molecules, respectively (4 °C, 20 min). For detection of tetramer-positive cells in blood, activated T cells were gated on high CD38-expression. Before flow cytometry acquisition, cells were labelled with 7-ADD to exclude dead cells and avoid unspecific staining. Statistical analyses Differences between mean values were assessed by Student’ t -test for single comparison or ANOVA for multiple comparisons. Student’s t -test was for paired or unpaired samples: the paired test was used to compare responses to antigen and controls in the same donor, the unpaired test was used to compare responses of psoriasis patients vs HD or control-patients responses. T tests for assessing proliferation to LL37, measured as stimulation indexes (SI, see below), were one-tailed and variance between HD and psoriasis patients was assumed to be inequal, as HD did not respond to LL37. Statistical significance was set at P <0.05. Correlation between PASI/intensity of LL37-specific primary responses (SIs) (proliferation/cytokine production) was assessed by Spearman rank-correlation test. SI for proliferation was calculated by dividing percent of BrdU-staining in the presence of each peptide by percent of BrdU staining in the absence of peptide stimulation. SI/cytokines was obtained by dividing values of cytokine secretion (measured by ELISA) in the presence of peptides by values of cytokine secretion in the absence of peptides. For IL-17 and IL-21, SI/cytokines was also obtained by dividing values of % of T cells that became positive for cytokine expression (measured by intracellular staining by flow cytometry) in the presence of peptides by values of % of T cells positive for cytokine expression in the absence of peptides. SI for proliferation was considered positive when >3. This cut-off was obtained by calculating the mean+2DS [1.5+2 (0.6)] (of the stimulation indexes calculated as above) of the proliferation of HD. The PASI was also correlated to mere positivity/negativity of LL37-specific primary T-cell proliferation/cytokine production. Positive responses for cytokines were those having SI/cytokines >2. For this correlation we used k statistics [29] , [70] providing values of +1 (perfect agreement) to –1 (complete disagreement) via 0 (no agreement above that expected by chance). How to cite this article: Lande, R. et al . The antimicrobial peptide LL37 is a T-cell autoantigen in psoriasis. Nat. Commun. 5:5621 doi: 10.1038/ncomms6621 (2014).